Ripple-modulated electronic structure of a 3D topological insulator Three-dimensional topological insulators host linearly dispersing states with unique properties and a strong potential for applications. An important ingredient in realizing some of the more exotic states in topological insulators is the ability to manipulate local electronic properties. Direct analogy to the Dirac material graphene suggests that a possible avenue for controlling local properties is via a controlled structural deformation such as the formation of ripples. However, the influence of such ripples on topological insulators is yet to be explored. Here we use scanning tunnelling microscopy to determine the effects of one-dimensional buckling on the electronic properties of Bi 2 Te 3. By tracking spatial variations of the interference patterns generated by the Dirac electrons we show that buckling imposes a periodic potential, which locally modulates the surface-state dispersion. This suggests that forming one- and two-dimensional ripples is a viable method for creating nanoscale potential landscapes that can be used to control the properties of Dirac electrons in topological insulators. The helical Dirac fermions that exist on the surface of topological insulators (TIs) are condensed matter analogues of relativistic fermions extensively studied in high-energy physics [1] , [2] , [3] , [4] , [5] , [6] . Many theoretical scenarios in high-energy physics such as Majorana fermions and axion electrodynamics are also anticipated to manifest experimental signatures in TIs [2] , [7] , [8] , [9] . The greatest challenge for achieving these and other exotic states is the ability to control properties such as electron mobility or the position of chemical potential with respect to the bulk bands. Controlling and manipulating these properties on a local scale is particularly important in TIs, where phase boundaries, dislocations and domain walls are predicted to have a special role. One possible method of engineering potential landscapes in TIs is via positioning dopants in a controlled fashion. Although bulk doping is difficult to manipulate, using surface dopants shown to result in global chemical potential shifts [10] , [11] , [12] , [13] remains a possible option. However, this method is not ideal for various reasons: First, surface doping has been shown to create multiple topologically trivial surface states that can complicate measurements [10] , [11] , [12] , [13] . Second, although doping can be used to create large changes in the spatially averaged chemical potential, using this method to manipulate the local potential is non-trivial [14] . Finally, although backscattering is forbidden in TIs, as demonstrated by Landau level measurements [15] , surface dopants have been shown to have a strongly detrimental effect on the electron coherence and lifetime [15] . As suggested by extensive studies on the Dirac material graphene, another avenue to modulate electronic properties on a local scale is via the creation of ripples, which has the tremendous advantage that the system remains chemically pristine. Experimentally, one-dimensional (1D) and two-dimensional (2D) periodic ripples have been created in graphene by the strain arising from clamped edges or due to an incommensurability with the growth substrate [16] , [17] , [18] . Theoretical models of ripples in graphene suggest that the resulting local surface curvatures affect the microscopic parameters of the electronic states such as hopping matrix elements and the coupled dispersion relations. In addition to changing microscopic parameters and creating local effects such as strong pseudomagnetic fields [19] , structural ripples can also result in an added periodic potential [20] in the energy landscape. The effects of such periodic potentials on the electronic structure of graphene have been extensively explored theoretically [21] , [22] , [23] , [24] , [25] where it was shown that periodic potentials may not only change band parameters similar to the Fermi velocity but also induce additional zero energy modes and bandgaps. However, while the charge and lattice degrees of freedom are intimately coupled in graphene, it is not clear a priori how a physical buckling from similar structural ripples might influence the surface and bulk band structure in TIs. Therefore, an essential first step in determining their viability in controlling the local electronic properties of TI's is the experimental mapping of the spatially resolved electronic structure of rippled TIs. In this work, we investigate the effects of a 1D periodic buckling and its associated chemical inhomogeneity on the electronic properties of the TI, Bi 2 Te 3 (ref. 26 ). We use low-temperature scanning tunnelling microscopy (STM) and spectroscopy, to probe the electronic structure of this surface. By carrying out local Fourier transforms (FTs) of the spatial maps of interference patterns, we clearly demonstrate that in contrast to the non-local effects of chemical dopants, buckling has a well-defined, local effect on the Dirac dispersion. Our studies suggest that generating ripples provides an avenue to engineer the potential landscape in TIs. Topography of rippled Bi 2 Te 3 STM images of Bi 2 Te 3 ( Fig. 1 ) reveal two kinds of regions: flat areas with no ripples and regions with a 1D periodic modulation, that is, stripes ( Fig. 1a ). Striped regions were observed with several tips and on various cleaved surfaces. The stripes have a periodicity of ~100 nm, ~0.1 nm height, and are aligned to within 5 degrees of ΓM (next-nearest neighbor) direction. Within one sample, the striped areas extend for at least a few micrometres and are adjacent to flat areas. On the basis of the topographic characteristics alone, the stripes may originate from a modulation of the atomic positions (buckling) or purely electronic modulations due to charge or spin density wave order. The large ~100 nm periodicity and the lack of contrast reversal at opposite bias voltages ( Fig. 1e-g ) is, however, inconsistent with a conventional electronic charge density wave or a pure charge inhomogeneity, indicating that the stripes represent spatial modulations in height. Although it is not explicitly clear which interactions [27] might produce these features, a probable explanation is that the buckling occurs during sample growth or cleaving due to strain. Strain for instance has been shown to result in a 1D reconstruction at various length scales and can affect both the lattice and the electronic structure [17] , [28] , [29] , [30] . Empirically, in the present study, we expect that strain causes a modulation of the height of the atoms perpendicular to the surface, resulting in the periodic buckling observed in the topography. 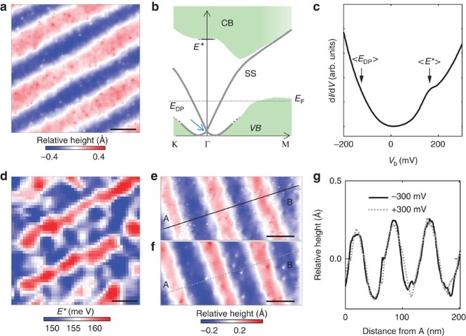Figure 1: Topography and variation of bulk conduction band across stripes in Bi2Te3. (a) Topography of stripes on the surface of Bi2Te3obtained with bias voltage (Vb) =+250 (mV). (b) A schematic of the band structure of surface and bulk bands (green area)34together with the approximate position of the Fermi energy (EF) in our samples. (c) Spatially averaged dI/dVspectrum in the region shown ina. The arrows show the approximate position for the Dirac point (EDP) and the bulk conduction band edge around Γ point,E*. The association of the resonance feature in the STM dI/dVspectra with the conduction band edge was determined in previous STM studies31,32,33. (d) Spatial map ofE*showing variations with stripes. (e,f) Topographic stripes atVb=+300 and −300 mV, respectively, showing the absence of contrast reversal at positive (e) and negative (f) biases. These images were obtained on a different sample from that shown ina. (g) Height variation across the lines shown in (e,f). The scale bars inaanddrepresent 60 nm, and those ineandfare 40 nm. arb. units increpresent arbitrary units. Figure 1: Topography and variation of bulk conduction band across stripes in Bi 2 Te 3 . ( a ) Topography of stripes on the surface of Bi 2 Te 3 obtained with bias voltage ( V b ) =+250 (mV). ( b ) A schematic of the band structure of surface and bulk bands (green area) [34] together with the approximate position of the Fermi energy ( E F ) in our samples. ( c ) Spatially averaged d I/ d V spectrum in the region shown in a . The arrows show the approximate position for the Dirac point ( E DP ) and the bulk conduction band edge around Γ point, E* . The association of the resonance feature in the STM d I/ d V spectra with the conduction band edge was determined in previous STM studies [31] , [32] , [33] . ( d ) Spatial map of E* showing variations with stripes. ( e , f ) Topographic stripes at V b =+300 and −300 mV, respectively, showing the absence of contrast reversal at positive ( e ) and negative ( f ) biases. These images were obtained on a different sample from that shown in a . ( g ) Height variation across the lines shown in ( e , f ). The scale bars in a and d represent 60 nm, and those in e and f are 40 nm. arb. units in c represent arbitrary units. Full size image Influence of buckling on the bulk bands STM spectra of Bi 2 Te 3 capture the density of states arising from the surface projection of the bulk bands as well as the Dirac surface states. A telltale feature in the spectroscopy is a broad resonance at higher energies, labelled E * in Fig. 1c , that has previously been identified as the energy of the bottom of the surface-projected conduction band at the Γ point as shown in Fig. 1b via a comparison between STM and angle-resolved photoemission spectroscopy data [31] , [32] , [33] , [34] . Tracking the energy of E * allows us to follow spatial shifts in the bulk bands with respect to the Fermi energy. A plot of the energy of E *, with position ( E * map) as shown in Fig. 1d , indicates that the E * values are modulated by the ripples. This correlation between the buckling and the bulk bands is also clearly observed in a 2D histogram of E * values plotted against relative height, which reveals a bimodal split ( Supplementary Fig. S1 ). On average, the value of E * is lower by ~10 meV in the region surrounding the crest of the stripes (higher region) compared with the region around the troughs ( Fig. 1d and Supplementary Fig. S1 ). These data indicate that the bulk bands in the crests are shifted in energy with respect to the bulk bands in the troughs by ~10 meV. Effect of ripples on the Dirac surface-state bands Prior studies have shown that in samples with random potential variations the local surface and bulk bands are shifted together (rigid-band shift) in response to the local potential [14] , and the question is whether the ripples cause a similar effect. To measure the effect of the stripes on the surface state, we obtain spatial differential conductance maps (d I/ d V ( r ,eV )) as a function of energy ( Fig. 2 ). A 2D FT ( Fig. 2c ) of the spatial map ( Fig. 2a ) at a given energy captures the scattering vectors ( q -vectors) that connect different points of the constant energy contour at that energy ( Fig. 2b ). This technique can be used to trace back to the original momenta ( k ) of the electrons and obtain the resulting dispersion. From previous STM studies [31] , [32] , [33] the dominant q -vector at higher energies in the high-symmetry direction is q ΓM , as depicted in Fig. 2b . To capture the spatial variation of q ΓM , we first carried out spatially resolved FTs of the conductance maps. The results are shown in Fig. 2d–f , which plots the spatially resolved q -vector magnitudes | q ΓM | and their average value ( Fig. 2g ). These q -maps were extracted from peak positions along ΓM of FTs of local patches (45×45 nm sized areas corresponding to ~0.015 (nm –1 ) resolution in momentum space). In contrast with previous studies showing no correlations between impurity density and electronic structure [14] , our spatially resolved FTs reveal an unambiguous correlation between the topography with striped corrugation and the dispersion of the Dirac surface states. Specifically, the magnitude of q ΓM systematically shows a larger value at the crest of the stripes. 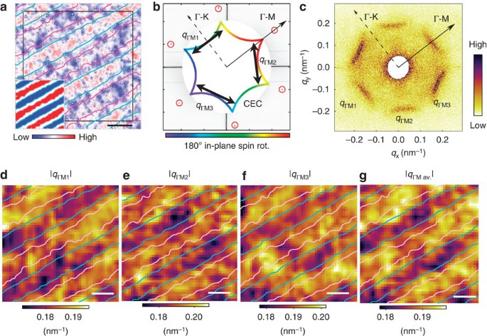Figure 2: Spatial map of local scattering vector along ΓM,qΓM. (a) dI/dV (r, eV) (conductance) map atVb=+250 mV in striped region shown inFig. 1a. The inset shows the red and blue regions used later inFig. 2. The regions were defined by dividing the total height of the ripples into three ranges: red (higher region around crest), white (middle) and blue (lower region around trough), with the constraint that the areas are the same and equal to 1/3 the total area. The lines (pink and light blue) define the boundaries of these three regions. (b) FT of topographic image shown inFig. 1a. The inset shows a schematic constant energy contour (CEC) at +250 mV (380 mV above the approximate spatially averaged Dirac point of −130 mV in these samples), displaying a snowflake-like shape. The schematic CEC is superimposed on the Fourier transform of the topography, which shows the Bragg peaks highlighted by red circles. (c) FT of the conductance map ina. The characteristicq-vectorsqΓM1,qΓM2andqΓM3connecting well-nested portions of the CECs shown schematically inbare clearly visible along the ΓM directions. (d–f) Spatial maps at +250 meV of local |qΓM1|, |qΓM2| and |qΓM3| obtained from 45 nm square patches and average value (g), for the area enclosed by the black square shown ina. The lines (pink and light blue) are defined as ina. The scale bar inais 60 nm and is 50 nm ind–f. Figure 2: Spatial map of local scattering vector along ΓM, q ΓM . ( a ) d I/ d V ( r , eV) ( conductance) map at V b =+250 mV in striped region shown in Fig. 1a . The inset shows the red and blue regions used later in Fig. 2 . The regions were defined by dividing the total height of the ripples into three ranges: red (higher region around crest), white (middle) and blue (lower region around trough), with the constraint that the areas are the same and equal to 1/3 the total area. The lines (pink and light blue) define the boundaries of these three regions. ( b ) FT of topographic image shown in Fig. 1a . The inset shows a schematic constant energy contour (CEC) at +250 mV (380 mV above the approximate spatially averaged Dirac point of −130 mV in these samples), displaying a snowflake-like shape. The schematic CEC is superimposed on the Fourier transform of the topography, which shows the Bragg peaks highlighted by red circles. ( c ) FT of the conductance map in a . The characteristic q -vectors q ΓM 1 , q ΓM 2 and q ΓM 3 connecting well-nested portions of the CECs shown schematically in b are clearly visible along the ΓM directions. ( d – f ) Spatial maps at +250 meV of local | q ΓM 1 |, | q ΓM 2 | and | q ΓM 3 | obtained from 45 nm square patches and average value ( g ), for the area enclosed by the black square shown in a . The lines (pink and light blue) are defined as in a . The scale bar in a is 60 nm and is 50 nm in d – f . Full size image The clear correlation between striped topography and q -maps motivates us to define distinct larger regions for our FTs. On the basis of the topographic height we separate the region into three areas with same coverage, that is, 1/3 of the total area ( Fig. 3 ), as per the inset in Fig. 2a . Selective FTs of these larger regions gives us better q -resolution, allowing us to track the energy dependence of the q -vectors and thereby measure the relative energy shift of the surface-state band. As we do not observe any systematic anisotropies in q -vector magnitude along the three equivalent directions in k -space, we consider the three q ΓM 's equivalent and perform our analysis on the symmetrized FTs shown in Fig. 3 . Similar to the previous study of doping-induced inhomogeneity, we find that there is a measureable difference between the q -vectors obtained in the crests (red) and troughs (blue) regions ( Fig. 3b–d ). In converting back to the originating momenta we plot the surface-state dispersion obtained from the interference patterns in Fig. 4 . 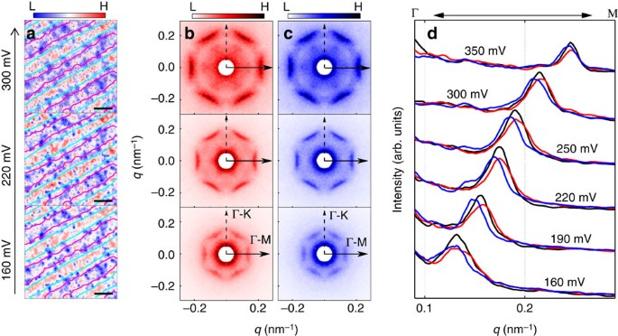Figure 3: Surface-state dispersion probed by standing wave patterns. (a) Conductance maps at +300, +220 and +160 mV (top to bottom). The lines define the boundaries of the high and low regions (red and blue) as shown in the inset ofFig. 2a. The scale bar is 60 nm. (b,c) FT of the red (b) and blue (c) regions, respectively. The FTs are sixfold symmetrized and have been rotated such that the ΓM direction is along thexaxis. (d) Energy dependence of the linecuts along ΓM of FT images from the lower (blue line), higher (red line) and all (black line) regions. Figure 3: Surface-state dispersion probed by standing wave patterns. ( a ) Conductance maps at +300, +220 and +160 mV (top to bottom). The lines define the boundaries of the high and low regions (red and blue) as shown in the inset of Fig. 2a . The scale bar is 60 nm. ( b , c ) FT of the red ( b ) and blue ( c ) regions, respectively. The FTs are sixfold symmetrized and have been rotated such that the ΓM direction is along the x axis. ( d ) Energy dependence of the linecuts along ΓM of FT images from the lower (blue line), higher (red line) and all (black line) regions. 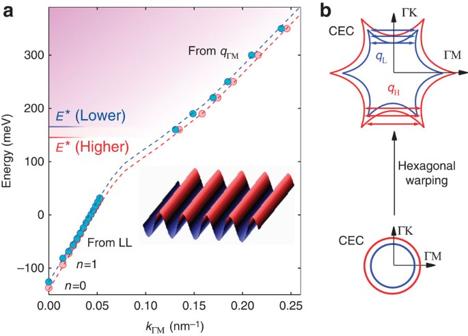Figure 4: Riple-modulated band dispersion. (a) Peak positions obtained from linecuts shown inFig. 3dtogether with data points from previously reported Landau level (LL) spectra atB=7T35. The dotted line is a guide to the eye and depicts the dispersion of the surface-state band along ΓM based on previous angle-resolved photoemission spectroscopy studies of Bi2Te3(ref.34) but rigidly shifted to match the position of our Fermi energy.E*values within the bands are based on the maximum and minimum value measures by us on the stripes. The inset shows a schematic rippled surface. The blue and red colours in the schematic as well as the symbols represent the topographically higher and lower regions, respectively. (b) Schematic constant energy contours based on our data for the topographically higher (red) and lower (blue) regions. The isotropic circles and snowflake-like shape represent the CECs close to the Dirac point and at higher energies, where LLs and intererence patterns shown in (a) were obtained, respectively.qHandqLdepict the scattering vectors along ΓM in the higher (red) and lower (blue) regions as ina. Full size image Figure 4: Riple-modulated band dispersion. ( a ) Peak positions obtained from linecuts shown in Fig. 3d together with data points from previously reported Landau level (LL) spectra at B =7T [35] . The dotted line is a guide to the eye and depicts the dispersion of the surface-state band along ΓM based on previous angle-resolved photoemission spectroscopy studies of Bi 2 Te 3 (ref. 34 ) but rigidly shifted to match the position of our Fermi energy. E* values within the bands are based on the maximum and minimum value measures by us on the stripes. The inset shows a schematic rippled surface. The blue and red colours in the schematic as well as the symbols represent the topographically higher and lower regions, respectively. ( b ) Schematic constant energy contours based on our data for the topographically higher (red) and lower (blue) regions. The isotropic circles and snowflake-like shape represent the CECs close to the Dirac point and at higher energies, where LLs and intererence patterns shown in ( a ) were obtained, respectively. q H and q L depict the scattering vectors along ΓM in the higher (red) and lower (blue) regions as in a . Full size image Role of impurities (inclusive of vacancies) in creating the periodic buckling and potential Next we examine the possible correlation between chemical disorder inhomogeneity and the observed electronic modulation. Although previous studies of random doping-induced inhomogeneity showed no spatial correlations between the dopant density and the potential variations, we find that there is a weak, positive correlation between the topography and the density of one of the impurity species, which can be identified as an electron donor ( Fig. 5 , also see Supplementary Figs S2–S4 , and Supplementary Discussion for further details including the methodology in calculating these correlations). This correlation ( C (0)=0.3), however, is far weaker than the correlation between the topography and electronic structure modulations as measured by the q -vector variations in the interference patterns as well as E * values ( C (0)=0.65) ( Fig. 5a ), suggesting that the small changes in the impurity density are likely a secondary effect. This is further supported by the equally strong on-site correlation between the topography and the n =1 Landau level energies ( Fig. 5a ), which directly reflects the varying potential due to the stripes. We therefore conclude that the potential variations originate from the ripples rather than any changes in impurity density. 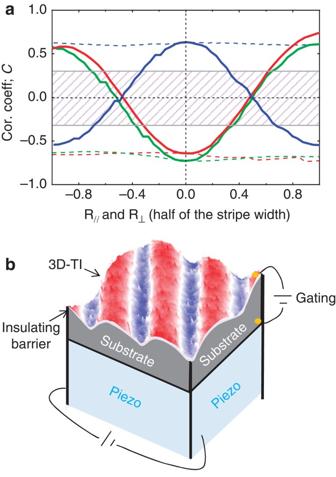Figure 5: Correlation between topograohic ripples and periodic potential. (a) Plot of the cross-correlation coefficients (cor. coeff.) between the topographic height (T(r)) and three spatially varying parameters: bulk band variation represented byE*(green line); surface-state band variation represented byqΓMat 250 mV aboveEF(blue line), and then=1 Landau level near the Dirac point (red line)35. These are plotted along the directions perperdicular (, solid lines) and parallel to the stripes (R//, dotted lines). The methodology for this calculation is in theSupplementary Information. The plot shows that the maximum correlation values are onsite atR//==0. The shaded area represents the maximum cor. coeff. of ~0.3 observed between impurity potentialφ2(r) and the three maps:E*(r),q(r) andT(r) (seeSupplementary Fig. S3andSupplementary Discussion). (b) Schematic of a possible stripe-based device with the stripes generated by the strain created by a piezoelectric crystal. Figure 5: Correlation between topograohic ripples and periodic potential. ( a ) Plot of the cross-correlation coefficients (cor. coeff.) between the topographic height ( T ( r )) and three spatially varying parameters: bulk band variation represented by E* (green line); surface-state band variation represented by q ΓM at 250 mV above E F (blue line), and the n =1 Landau level near the Dirac point (red line) [35] . These are plotted along the directions perperdicular ( , solid lines) and parallel to the stripes ( R // , dotted lines). The methodology for this calculation is in the Supplementary Information . The plot shows that the maximum correlation values are onsite at R // = =0. The shaded area represents the maximum cor. coeff. of ~0.3 observed between impurity potential φ2 ( r ) and the three maps: E* ( r ), q ( r ) and T ( r ) (see Supplementary Fig. S3 and Supplementary Discussion ). ( b ) Schematic of a possible stripe-based device with the stripes generated by the strain created by a piezoelectric crystal. Full size image From the data shown in Fig. 4a we find that the surface-state dispersion in the crests of the stripes is shifted to higher energies by ~10 meV compared with that in the troughs of the stripes. In addition, Landau level measurements across the stripes show that the lower index ( n =0 and 1) [35] levels faithfully track the higher energy dispersion obtained from the interference patterns, proving that the electrons close to the Dirac point are equally affected by the stripes. Moreover, this energy scale is consistent with the shift observed for the bulk bands from E * shown in Fig. 1 ; all of which indicate that the stripes create a 1D periodic potential landscape that affects the bulk and surface-state bands in a similar fashion. The picture that emerges from our data is the following: The periodic buckling represented by the stripes results in a smoothly varying periodic potential that is primarily responsible for trapping the carriers into the resultant 1D potential wells and shifting the bulk and surface states bands according to a rigid-band shift picture. An intriguing consequence of our observations is that in a magnetic field, such periodic chemical potential variations can play host to 1D chiral metallic modes. Analogous to edge states in an integer quantum Hall system, 1D modes are predicted at the spatial boundaries between two regions with successive half-integer fillings [2] , [6] . These modes are interesting as practical realizations of 1D quantum wire states and can potentially be used to achieve dissipationless transport in 1D ( Fig. 5b ). Finally, our studies clearly show that for TIs creating ripples is an efficient method for manipulating electronic properties on a local scale. We stress here that even though the stripes in these studies have not been generated in a controlled fashion, our results provide an essential first step for exploring the viability of strain engineering TIs. It would be worthwhile to explore the generation of similar ripple features by annealing and quenching of bulk crystals, inducing strain in thin films with substrate mismatch, or by actively induced strain via piezo actuators. Materials The single crystals of Bi 2 Te 3 used in this study were grown via a standard modified Bridgman method [36] . Bulk transport measurements show that the sample is p-type as expected. The crystal surface was obtained by cleaving in ultrahigh vacuum at room temperature before being inserted into the STM held at 4 K. Measurements Tungsten tips prepared by flash annealing were used in this study. d I /d V spectra and maps (conductance maps) were obtained with a lock-in amplifier. How to cite this article: Okada, Y. et al . Ripple-modulated electronic structure of a 3D topological insulator. Nat. Commun. 3:1158 doi: 10.1038/ncomms2150 (2012).